Evidence for charge–vortex duality at the LaAlO3/SrTiO3interface The concept of duality has proved extremely powerful in extending our understanding in many areas of physics. Charge–vortex duality has been proposed as a model to understand the superconductor to insulator transition in disordered thin films and Josephson junction arrays. In this model, on the superconducting side, one has delocalized Cooper pairs but localized vortices; while on the insulating side, one has localized Cooper pairs but mobile vortices. Here we show a new experimental manifestation of this duality in the electron gas that forms at the interface between LaAlO 3 and SrTiO 3 . The effect is due to the motion of vortices generated by the magnetization dynamics of the ferromagnet that also forms at the same interface, which results in an increase in resistance on the superconducting side of the transition, but an increase in conductance on the insulating side. The two-dimensional superconductor to insulator transition (SIT) has been studied extensively [1] , [2] , [3] , as experimentally it is one of the few easily accessible manifestations of a quantum phase transition. The two-dimensional electron gas formed at the LaAlO 3 /SrTiO 3 (LAO–STO) interface [4] , [5] , [6] has been shown to undergo a SIT as the density of the carriers is tuned [7] , [8] , [9] . In addition to superconductivity, our earlier work showed evidence of ferromagnetism, which manifests itself as a hysteresis in measurements of the magnetoresistance (MR), Hall effect and superconducting phase boundary [8] . Two other recent studies have confirmed the coexistence of superconductivity and magnetism in similar samples [10] , [11] . Theoretical calculations suggest that the magnetism arises from localized moments on Ti ions at the interface [12] . Ferromagnetic order is stablized via RKKY interactions mediated by the conductance electrons. The experimental evidence obtained so far [8] , [10] indicates that the effect of the ferromagnetism on the electrical transport properties of the system can be accounted for by considering only the magnetic field produced by the ferromagnet. In this paper, we show that the coexistence of ferromagnetism and superconductivity in this system leads to a novel manifestation of charge–vortex duality in the SIT. On the superconducting side of the transition, the dynamics of the ferromagnet during magnetization reversal leads to a sharp peak in resistance whose magnitude increases with the sweep rate of the magnetic field. On the insulating side of the transition, the same magnetization dynamics lead to a dip in resistance whose magnitude again increases with the magnetic field sweep rate. This behaviour can be understood by modelling the superconductor as a random network of superconducting islands that responds to the dynamic magnetic field arising from the ferromagnet. MR in the superconducting state The samples in this work had 10 unit cells (uc) of LAO grown by pulsed laser deposition on TiO 2 -terminated (001) STO single-crystal substrates [13] , [14] . Details of sample fabrication were discussed in an earlier publication [8] (see also Methods). The interaction between ferromagnetism and superconductivity can be seen in MR measurements in the superconducting state. 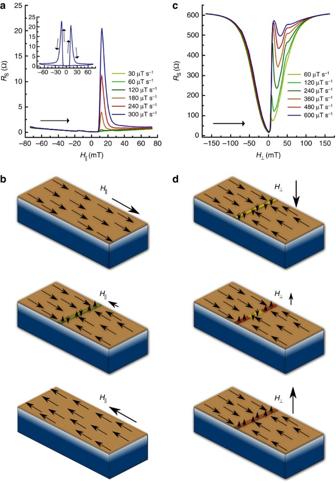Figure 1: MR in the superconducting regime. (a) Parallel field MR as a function of different rates in the superconducting regime atVg=80 V. Data for only one field sweep direction are shown for clarity. Arrow indicates the direction of field sweep. The inset shows the MR for forward and backward field sweep directions at a sweep rate of 300 μT s−1. (b) Schematic of the system at different parallel field values. The top layer is the ferromagnet, the superconductor is shown through a gradient as extending some distance into the STO. In this simplified picture, magnetization reversal occurs by means of domain wall propagation in the ferromagnet. The perpendicular component of the field due to the domain wall induces vortices in the superconductor. (c) Perpendicular field MR for fields swept from negative to positive values for different field sweep rates forVg=80 V. (d) Schematic of the magnetization state of the system at different perpendicular fields. Owing to the shape anisotropy of the system, the majority of the moments lie in plane, but the external magnetic field orients the direction of the perpendicular component of the magnetization of the domain wall. It should be emphasized that the magnetization configuration in the real system during reversal is definitely far more complicated, but would still give rise to a perpendicular component of the magnetic field. All data were taken atT=50 mK. Figure 1 shows the MR in a magnetic field parallel and perpendicular to the plane of the sample, respectively, at T= 50 mK and V g =80 V, a gate voltage at which the sample is maximally superconducting. Consider first the case of a parallel magnetic field, H || ( Fig. 1a ). As has been seen earlier for this sample in perpendicular magnetic fields [8] , the parallel field MR is hysteretic due to the presence of ferromagnetic order (inset of Fig. 1a ). As H || is in the plane of the two-dimensional superconductor, the critical field is large (see Methods), so that one expects the MR to be small in this field range. In fact, the overall background MR is indeed quite small: most of the contribution to the MR is due to a set of twin peaks at ±12 mT. For clarity, we show in Fig. 1a the MR for only one sweep direction. As H || is increased from negative values, there is a small decrease in the resistance of the sample until H || =0. The peak in the MR develops just as H || becomes positive for this field sweep direction, but then rapidly dies out as H || is increased further. The most surprising fact about the MR of Fig. 1a is that the amplitude of the peak depends on the sweep rate of H || : the amplitude increases as the field sweep rate is increased. For very slow sweep rates, the peak is almost absent, and the amplitude of the overall MR is very small, as expected from our earlier discussion. Figure 1: MR in the superconducting regime. ( a ) Parallel field MR as a function of different rates in the superconducting regime at V g =80 V. Data for only one field sweep direction are shown for clarity. Arrow indicates the direction of field sweep. The inset shows the MR for forward and backward field sweep directions at a sweep rate of 300 μT s −1 . ( b ) Schematic of the system at different parallel field values. The top layer is the ferromagnet, the superconductor is shown through a gradient as extending some distance into the STO. In this simplified picture, magnetization reversal occurs by means of domain wall propagation in the ferromagnet. The perpendicular component of the field due to the domain wall induces vortices in the superconductor. ( c ) Perpendicular field MR for fields swept from negative to positive values for different field sweep rates for V g =80 V. ( d ) Schematic of the magnetization state of the system at different perpendicular fields. Owing to the shape anisotropy of the system, the majority of the moments lie in plane, but the external magnetic field orients the direction of the perpendicular component of the magnetization of the domain wall. It should be emphasized that the magnetization configuration in the real system during reversal is definitely far more complicated, but would still give rise to a perpendicular component of the magnetic field. All data were taken at T =50 mK. Full size image The rate dependence of the MR can be understood if we consider the influence of the domain wall of the ferromagnet on the superconductor, as shown schematically in Fig. 1b . In the simplest model, as H || is swept from a large negative to a large positive value, the magnetization of the ferromagnetic layer reverses by forming a domain wall that propagates from one end of the sample to the other once H || >0. If the domain wall is a Bloch wall [15] , the magnetization points out of the plane of the interface, and the conducting layer sees a magnetic field perpendicular to the interface that is localized near the domain wall, and travels along with it. We emphasize that for the real sample, the magnetization dynamics are likely far more complicated, but the end result of a localized magnetic field perpendicular to the plane of the interface that moves as H || is swept is the same. At the field sweep rates in the experiment, the motion of the domains is quasi-static. Consequently, the motion of the localized perpendicular magnetic field is determined only by the sweep rate of the external magnetic field. The moving perpendicular component of the field in turn generates moving vortices in the superconductor. For our samples, which can be thought of as granular superconductors (see below), moving vortices will result in a change in resistance [16] as the vortices cross the weak links between superconducting grains. Similar behaviour is also observed for the MR in a perpendicular external magnetic field ( Fig. 1c ). Given the two-dimensional nature of the ferromagnet [12] , it is unlikely that the perpendicular magnetic fields applied can cant the moments appreciably out of plane. However, a Bloch domain wall may form at the interface, and it is domains within this Bloch wall that are reoriented in an external magnetic field, as shown in Fig. 1d . Such behaviour has been seen before in thin magnetic films [17] . (We stress again that this picture is highly simplified, and the real reversal process is likely much more complicated.) itself leads to a large overall MR, with a minimum at zero field. The field from the ferromagnet gives rise to a sweep rate–dependent peak at ~±15 mT, and a second, less prominent peak at ~±48 mT, which is likely due to more complex magnetization dynamics in perpendicular field. Further evidence that the hysteresis and the dips are due to magnetization dynamics in the ferromagnet can be seen from the MR in crossed parallel and perpendicular fields. When one measures the background MR in a perpendicular field in the presence of a large constant parallel field that aligns the magnetization of the ferromagnet, no hysteresis or rate dependence is observed (see Methods). MR in the insulating state In the LAO/STO interface system, the superconducting transition can be tuned by V g (refs 7 and 8 ). Early studies of LAO/STO interfaces identified this as a SIT [7] , which has been studied extensively in the past in thin superconducting films as a function of the film thickness or an applied magnetic field [1] , [2] . However, in the LAO/STO system, it appears difficult to tune the system deep into the insulating regime with a gate voltage [9] . Nevertheless, measurements of the current-dependent differential resistance (Methods) indicate that the transition is to a weakly insulating state where regions of superconductivity get increasingly isolated from one another as V g is decreased. Thus, it makes sense to model our sample as a granular superconductor consisting of a network of superconducting islands whose phase is coupled through the Josephson effect, parametrized by the Josephson energy E J and a Coulomb charging energy E c , which is associated with the energy cost of adding a Cooper pair to an island [3] , [18] . (For a random network of islands, these quantities are averages over the network.) Changing V g in our sample tunes the transition by modifying the ratio between E J and E c . The superconducting and insulating regimes are duals of each other, and this duality is predicted to manifest itself through an interchange between specific measurable quantities [18] , [19] , [20] , [21] . For example, the current I and voltage V are interchanged across the SIT, so that the I – V curve in the superconducting phase is similar in shape to the V – I curve in the insulating state. Such dual I – V characteristics have been observed in Josephson junction arrays and disordered thin films [3] , [22] , [23] . In our samples, as noted above, it appears difficult to tune the system deep into the insulating regime, so that observing this signature of charge–vortex duality is difficult [6] , [8] . However, the interplay between ferromagnetism and superconductivity at the LAO/STO interface results in a unique manifestation of charge–vortex duality associated with moving ferromagnetic domain walls that has not been observed in other systems. 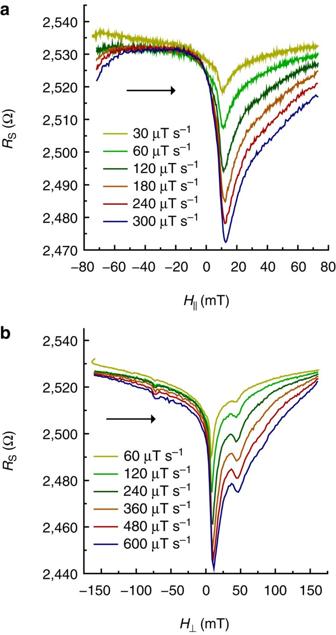Figure 2: MR in the insulating regime. (a) Parallel field MR forVg=−100 V. Data for only one field sweep direction are shown for clarity. Arrow indicates the direction of field sweep. (b) Perpendicular field MR forVg=−100 V.T=50 mK. Figure 2a,b demonstrates this new behaviour. Figure 2a shows the equivalent of the data of Fig. 1a , but at a gate voltage of V g =−100 V, placing the sample on the insulating side of the transition. At the same magnetic fields at which a sweep rate–dependent peak was seen in Fig. 1a , a sweep rate–dependent dip is observed. As with the peak, the magnitude of the dip increases with increasing sweep rate. Similar behaviour is observed in perpendicular magnetic field ( Fig. 2b ). Note that in perpendicular field, one even observes two sets of dips (at ±15 and ±48 mT), mirroring the behaviour seen in Fig. 1c . In the charge–vortex duality model, current and voltage are switched in going across the SIT, so that conductance and resistance are also switched. Thus, where one observes peaks in resistance on the superconducting side, one should observe peaks in conductance (or dips in resistance) on the insulating side. This is exactly what is observed. Figure 2: MR in the insulating regime. ( a ) Parallel field MR for V g =−100 V. Data for only one field sweep direction are shown for clarity. Arrow indicates the direction of field sweep. ( b ) Perpendicular field MR for V g =−100 V. T =50 mK. Full size image Gate voltage dependence of the peaks/dips As V g is changed from +80 to −100 V, tuning the system through the SIT, the peaks in the MR change to dips, as shown in Fig. 3a,b . A more striking graphical demonstration of the SIT can be seen if we plot the rate dependence of the resistance at the peaks or dips at different gate voltages normalized to their values at the highest sweep rate ( Fig. 4a,b ). The transition from peaks to dips in Figs 3 and 4 occurs at exactly the same V g as the transition from the superconducting to the insulating state in the R versus T dependence [8] . Thus the same phenomenon, that of magnetization dynamics in the ferromagnet, which causes an increase in resistance on the superconducting side, causes an increase in conductance on the insulating side. This interchange of resistance and conductance between the two different ground states of the system demostrates the duality of the two states. We note, however, that the resistance per square, R S , at which the transition occurs is approximately 2.1 kΩ, less than the universal resistance value of h /4 e 2 ~6.45 kΩ expected for the SIT [20] . 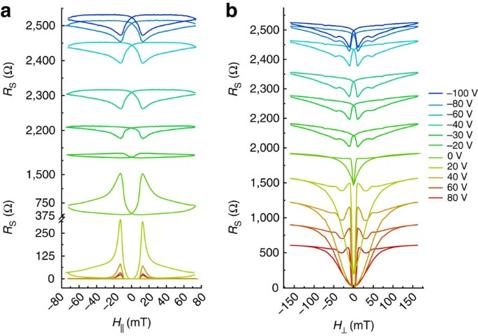Figure 3: SIT in the magnetoresistance. (a) Parallel field MR for the fastest sweep rate (300 μT s−1) as a function of gate voltage, tuning the system from the superconducting to the insulating regime. The top and bottom panels are for insulating and superconducting regimes, respectively. Charge–vortex duality manifests itself as the conversion of thepeakin the superconducting regime to adipin the insulating regime. The peak and dip occur at the external field value ofH||~±12 mT. (There is an axis break on theyaxis in the bottom panel.) The maximum change in the resistance occurs forVg=0 V, where the superconductivity is very weak. (b) Similar behaviour in perpendicular field. Note that the fastest sweep rate in this case is 600 μT s−1. Additional structure in the perpendicular field at~±48 mT is due to the more complex magnetization dynamics in the perpendicular field.T=50 mK. Figure 3: SIT in the magnetoresistance. ( a ) Parallel field MR for the fastest sweep rate (300 μT s −1 ) as a function of gate voltage, tuning the system from the superconducting to the insulating regime. The top and bottom panels are for insulating and superconducting regimes, respectively. Charge–vortex duality manifests itself as the conversion of the peak in the superconducting regime to a dip in the insulating regime. The peak and dip occur at the external field value of H || ~±12 mT. (There is an axis break on the y axis in the bottom panel.) The maximum change in the resistance occurs for V g =0 V, where the superconductivity is very weak. ( b ) Similar behaviour in perpendicular field. Note that the fastest sweep rate in this case is 600 μT s −1 . Additional structure in the perpendicular field at ~±48 mT is due to the more complex magnetization dynamics in the perpendicular field. T =50 mK. 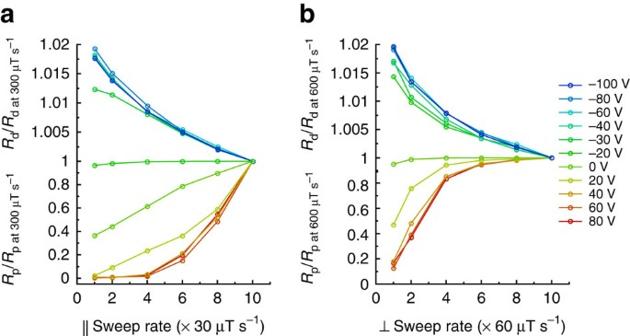Figure 4: Sweep rate dependence. (a) The evolution of the normalized resistance of the peaks and dips atH||~12 mT, with external field sweep rate as a function of the gate voltage for parallel field. The top and bottom panels are for insulating and superconducting regimes, respectively. (b) Similar plot for perpendicular field. The resistance of the peaks quickly saturates in the superconducting regime due to the additional pair breaking effect of the external field, unlike in the parallel field case.T=50 mK. Full size image Figure 4: Sweep rate dependence. ( a ) The evolution of the normalized resistance of the peaks and dips at H || ~12 mT, with external field sweep rate as a function of the gate voltage for parallel field. The top and bottom panels are for insulating and superconducting regimes, respectively. ( b ) Similar plot for perpendicular field. The resistance of the peaks quickly saturates in the superconducting regime due to the additional pair breaking effect of the external field, unlike in the parallel field case. T =50 mK. Full size image The peaks in the MR on the superconducting side are due to the magnetic field associated with a moving perpendicular component of the magnetization in the ferromagnet as the external magnetic field is swept. Given the fact that the position of the peaks and dips coincide for both and H || , it is clear that the dips also have the same origin. How would this field give rise to an increase in conductance on the insulating side? If the non-superconducting regime was simply a weakly localized metal, it would be hard to explain the dips in the MR that we observe (for a discussion, see Supplementary methods , which also contains alternate explanations of the MR dips, and why they do not account for our observations). These dips can be explained if one models the insulating side of the transition as one where the Cooper pairs are localized on isolated superconducting islands, and a Cooper pair requires an energy E c to transfer between two neighbouring islands, even though E c might be very small. Classically, the time-dependent magnetization of the ferromagnet gives rise to a time-dependent magnetic field, which in turn gives rise to an electric field =− ∂A / ∂t through Faraday's law; here A is the vector potential associated with the field. The voltage difference V =− d generated between two neighbouring superconducting islands separated by a distance d can exceed the charging energy E c , V > E c /2 e , so that the conductance of the system is momentarily increased. This explains the dips in MR in the insulating regime ( Fig. 3a,b ) when the domain wall passes through the ferromagnet. As we saw above, modelling our system as a granular superconductor explains the MR data qualitatively in both the superconducting and the insulating regimes. A more quantitative understanding of the peaks and dips can be obtained if one considers a thermal activation model for vortex motion in the superconducting regime and for charge transport in the insulating regime. As before, we begin with a discussion of the MR in the superconducting state. On the superconducting side of the transition, there is strong Josephson coupling between the islands ( E J E c ), and in the absence of motion of magnetic vortices, the sample is in the zero resistance state. Any magnetic vortices present exist in the interstitial regions between the islands. Motion of the magnetic vortices, which in our case is induced by the magnetization dynamics in the ferromagnet, will give rise to a finite resistance as the vortices cross the junctions between the superconducting islands. To understand the mechanism of the generation of this resistance, we use the phase slip model due to Langer and Ambegaokar (LA) [24] . There are corrections to this model, for example by McCumber and Halperin [25] , but the basic concepts are all that are essential for our analysis. For simplicity, we consider two adjacent superconducting islands that are Josephson coupled to each other at two points, so that the interstitial region between them can enclose a magnetic vortex: the sample consists of a network of such interconnected islands. (More generally, one probably has multiple interconnected islands enclosing vortices, but this does not change the physical picture.) These two islands can be thought of as a dc SQUID, whose energy profile is given by U ( )=− E J cos , where is the phase difference across the SQUID and E J is the Josephson energy. E J is proportional to the critical current I c of the SQUID. This defines a periodic potential where the minima of the potential correspond to integral values of the phase =2 n π. At finite temperature, the system can be thermally activated over the energy barrier represented by E J from one potential minimum to an adjacent minimum which differs by a value Δ =±2π. Each such phase slip event will give rise to a voltage pulse according to the Josephson relation , where the phase change is ±2π. In the absence of an external current, phase jumps in either direction are equally likely, hence the average voltage measured across the junction is zero, although such phase slip events may give rise to voltage noise. In the presence of an external measuring current I , the SQUID's energy profile is modified to the 'tilted washboard' potential . In this case, phase slip events corresponding to the system travelling 'down' the washboard tilt are slightly more likely than those in the other direction, leading to a finite average voltage, and hence a finite resistance. However, the probability of such events is still quite small at low temperatures if I I c . LA's original paper focused on phase slips in a single weak link between two superconductors. They derived the rate at which phase slips occur in each direction where the attempt frequency Ω depends on microscopic parameters as well as external parameters of the circuit. Here Δ F ± is the free energy barrier for phase jumps in the two directions [26] In the LA model, the application of a voltage V drives the generation of phase slips, and in steady state, the average voltage due to the generation of phase slips is equal to the applied voltage, giving the relation In the low current limit ( ) the corresponding resistance is In our case, a phase slip is generated whenever a magnetic vortex line crosses a weak link. The rate at which these phase slips are generated is then proportional to the time dependence of the field generated by the magnetization of the ferromagnet. At the field sweep rates in our experiment, the magnetization change is essentially quasi-static, hence this rate is proportional to the external magnetic field sweep rate , resulting in an additional factor in equation (4) proportional to . The change in resistance due to the motion of vortices for the entire sample is an average of terms such as equation (4) with a distribution of E J 's, but will be proportional to the magnetic field sweep rate . On the other hand, the measured value of the critical current I c of the sample will be determined by a parallel combination of random paths through the weak links connecting the superconducting islands. Nevertheless, it is reasonable to assume that this measured critical current I c is proportional to the mean Josephson energy E J for the superconducting network. Thus, we can write the change in resistance due to the motion of magnetic vortices in the form where I c is the measured critical current, and A and α are numerical constants at a fixed temperature. Thus, if one plots ln(Δ R ) as a function of I c at a fixed temperature, one should obtain a straight line. I c in this system can be varied by changing the gate voltage V g . 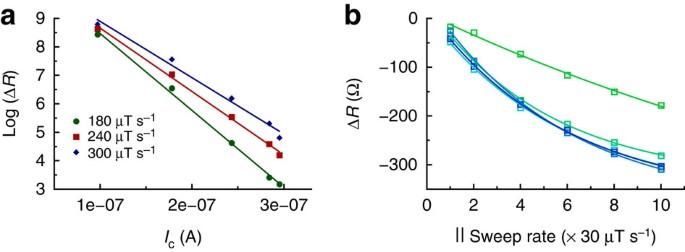Figure 5: Thermal activation model for the peaks/dips. (a) Log(ΔR) versusIcin the superconducting regime for the three fastest sweep rates in parallel external field. ΔRis defined as the difference in resistance between the forward and reverse magnetic field sweep traces atH||~12 mT. The five gate voltages corresponding to the fiveIcareVg=0, 20, 40, 60 and 80 V from the smallest to the largestIc. The three lines are the fits to the data at the three different sweep rates. (b) ΔRas a function of the parallel field sweep rate in the insulating regime. The data for each gate voltage,Vg=−30, −40, −60, −80 and −100 V, are fitted to an exponentially decaying function. Fitting parameters are given in the Discussion section.T=50 mK. Figure 5a shows this plot. As can be seen, the expected exponential dependence is indeed observed for a number of different magnetic field sweep rates. The slopes (equal to the exponential factor α/ k B T ) of the linear fits in Fig. 5a are 2.7×10 7 , 2.22×10 7 and 1.97×10 7 A −1 , for the three sweep rates, 180, 240 and 300 μT s −1 , respectively. The slopes (which should be equal for the three sweep rates) match to within about 25%. Figure 5: Thermal activation model for the peaks/dips. ( a ) Log(Δ R ) versus I c in the superconducting regime for the three fastest sweep rates in parallel external field. Δ R is defined as the difference in resistance between the forward and reverse magnetic field sweep traces at H || ~12 mT. The five gate voltages corresponding to the five I c are V g =0, 20, 40, 60 and 80 V from the smallest to the largest I c . The three lines are the fits to the data at the three different sweep rates. ( b ) Δ R as a function of the parallel field sweep rate in the insulating regime. The data for each gate voltage, V g =−30, −40, −60, −80 and −100 V, are fitted to an exponentially decaying function. Fitting parameters are given in the Discussion section. T =50 mK. Full size image Equation (5) also predicts that the resistance change should be proportional to the magnetic field sweep rate . If one looks at the parallel field data for V g =0 and 20 V shown in Fig. 4a , one can see that the dependence on sweep rate is indeed approximately linear. However, for V g =40, 60 and 80 V, which are deeper in the superconducting regime, the dependence is clearly not linear. In fact, deep in the superconducting regime, one might expect very little change in resistance, as the exponential factor involving I c in equation (5) would suppress any resistance change. Thus, the data at the three slowest sweep rates are not surprising. However, at higher sweep rates, the peak amplitude for these gate voltage values does increase. We do not know the reason for this, although one possibility is that at higher sweep rates, the effective Josephson coupling between islands is modified. We note that the data for the perpendicular field shown in Fig. 4b do not show a linear behaviour, but in this case, the situation is complicated by the fact that there is also a orbital contribution to the peak height due to the external perpendicular magnetic field. On the insulating side of the transition, a thermal activation model for charge transport can be developed in analogy with the vortex hopping model on the superconducting side. In this model, the rate at which charge can be transferred between islands is proportional to (ref. 27 ), and as with the superconducting regime above, charge transfers in both directions are equally likely, so there is no net average current. In the presence of a finite voltage difference Δ V between the two islands, the rate is modified to , and consequently favours charge transfer from the island at higher potential to the island at lower potential, resulting in a net average current between the islands. In our model, the potential Δ V results from the electric field that is generated by the moving magnetic field generated by the magnetization dynamics in the ferromagnet through Faraday's law. The time dependence of the changing magnetization, as we have pointed out above, is proportional to the sweep rate of the external magnetic field , and hence Δ V = γ , where γ is a constant. Thus, the resistance of the dip should have a dependence on the magnetic sweep rate of the form We note that this is a characteristically different dependence than that which is predicted and found in the superconducting regime. Figure 5b shows a plot of the resistance change at the dip as a function of the sweep rate for different gate voltages on the insulating side: the lines are fits to the exponential form, equation (6). As can be seen, the fits are quite good. The fit parameters for V g =−30, −40, −60, −80 and −100 V are, respectively: A =568.59, 332.77, 371.9, 381.05 and 373.59 Ω; B =578.56, 360.572, 379.10, 424.60 and 391.51 Ω; and k B T /γ=25.11, 5.22, 5.97, 5.79 and 5.89 μT s −1 . For V g =−100, −80, −60 and −40 V, the value of γ is almost the same. For V g =−30 V, it is quite different. The time-dependent magnetic field generates an electric field; the resulting voltage Δ V is proportional to the the electric field, but also to the spacing a between the islands. Hence γ should also depend on a . As V g is changed to bias the system closer to the transition from the insulating side, it is reasonable to expect that the effective spacing between islands decreases, resulting in a decrease in γ, as is observed in Fig. 5b . In summary, the LAO/STO interface, with its unusual combination of superconductivity and ferromagnetism, provides a unique signature of charge–vortex duality in the SIT. It would be interesting to see if similar signatures can be observed in artificially fabricated hybrid ferromagnet–superconductor structures. Experimental techniques The samples in this work had 10 unit cells (uc) of LaAlO 3 grown by pulsed laser deposition on TiO 2 -terminated (001) SrTiO 3 single-crystal substrates [13] , [14] . The electrical measurements were performed on a Hall bar defined by photolithography and etched using argon ion milling. Details of the film preparation, characterization and sample fabrication have been discussed in detail in previous publications [8] , [13] , [14] . The samples were measured in an Oxford dilution refrigerator with a base temperature of 15 mK. This refrigerator was equipped with a two-axis magnet so that a magnetic field could be applied both perpendicular and parallel to the LAO/STO interface. A gate voltage V g was applied to the back of the 500-μm-thick STO substrate. Transport measurements were made by a standard ac lock-in detection method. The samples were current biased with an excitation current of I ac =10 nA at a frequency of 11.3 Hz. For V g =20 V and higher, this excitation current is much less than the critical current, I c ( I ac <0.1 I c ). The voltage signals were first amplified using a low-noise homemade instrumentation amplifier and then measured using a PAR 124 analogue lock-in amplifier or an EG&G 7260 digital lock-in amplifier. Determination of film thickness and parallel critical field From the continuous mapping of T c versus one can estimate the superconducting coherence length, ξ , as discussed in ref. 8 . We obtained a value for the coherence length of ξ ~70 nm at V g =80 V. To determine the thickness of the superconducting layer, we performed a similar measurement of the dependence of T c on H || . The system was biased at the mid-point of the resistive transition ( R S =288 Ω at V g =80 V), under a proportional-integral-differential (PID) feedback circuit. The PID output was used to drive the mixing chamber heater while the field was ramped. This ensured that we always stayed at T c , defined as the mid-point of the resistive transition. A plot of T c versus H || measured in this way is shown in Fig. 6 . As expected for a two-dimensional superconductor, the dependence of T c on a parallel applied field is quadratic, except at low fields where hysteresis due to the ferromagnet suppresses T c . 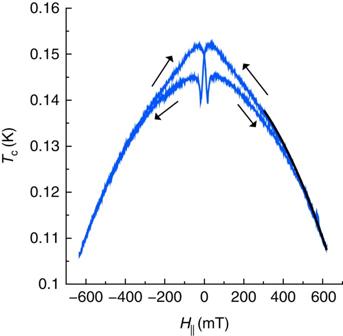Figure 6: Parallel critical field:TcversusH||forVg=80 V. A parabolic fit (black curve) at high fields givesHc||~1.2 T. The thickness of the superconducting layer estimated from this value isd=13.6 nm. From a fit to this measurement at high fields, we extracted the parallel critical field, H c|| ~ 1.2 T. For a thin film superconductor, H c|| and the film thickness are related by the formula [28] Figure 6: Parallel critical field: T c versus H || for V g =80 V. A parabolic fit (black curve) at high fields gives H c|| ~1.2 T. The thickness of the superconducting layer estimated from this value is d =13.6 nm. Full size image where Φ o = h /2 e is the superconducting flux quantum. From a knowledge of ξ and H c|| , we determined the thickness of the superconducting film to be d =13.6 nm, which is less than ξ . MR in crossed parallel and perpendicular fields As our system shows hysteresis due to the magnetization dynamics of the ferromagnet, it becomes inherently more complex to study the effect of an externally applied field to the system. To eliminate the hysteresis we applied a persistent parallel field, H || , which saturated the magnetization of the ferromagnet in one direction, and then performed perpendicular field MR measurements. In Fig. 7a , we show data in which perpendicular MR is measured for various values of H || for V g =100 V at T =50 mK. It can be seen that for H || =20 mT and higher, the sharp resistance peak in the MR is absent and the magnetization of the ferromagnet is completely saturated. For H || =0 mT, the sharp peak is recovered. Note that the minimum of resistance and the field at which this minimum occurs both increase as the parallel field is increased. The additional pair breaking caused due to a constant parallel field gives rise to the small increase in resistance. The shifting of the zero of the magnetic field is due to a small misalignment of plane of the sample with respect to the axis of our split coil magnet. From the shift we calculate the misalignment to be 1.4°. 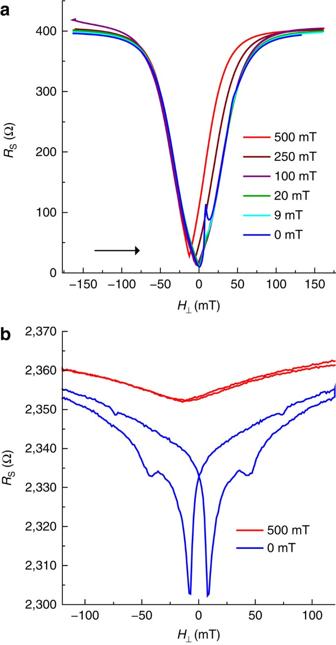Figure 7: Crossed parallel and perpendicular fields. (a)RSversusfor different values of parallel fields atVg=100 V. For clarity, field sweeps in only one direction are shown, with the arrow indicating the direction of field sweep. (b)RSversusforH||=0 and 500 mT atVg=−40 V. For both curves, the field is swept at the same rate of 120 μT s−1. ForH||=500 mT, characteristic features due to the ferromagnet are absent.T=50 mK for both the curves. Figure 7: Crossed parallel and perpendicular fields. ( a ) R S versus for different values of parallel fields at V g =100 V. For clarity, field sweeps in only one direction are shown, with the arrow indicating the direction of field sweep. ( b ) R S versus for H || =0 and 500 mT at V g =−40 V. For both curves, the field is swept at the same rate of 120 μT s −1 . For H || =500 mT, characteristic features due to the ferromagnet are absent. T =50 mK for both the curves. Full size image In the insulating phase (for V g =−40 V, say) the generation of flux due to domain wall motion is responsible for a rise in conductance. As discussed above, a changing vector potential, , generates an electric field, ɛ H , which causes a potential, V , to develop between two adjacent islands. When this potential energy 2 eV exceeds the charging energy of the islands, E c , one gets conduction between the islands. To see that the dips in resistance that we see on the insulating side are indeed due to such a mechanism, we show R versus traces for V g =−40 V, for H || =0 and 500 mT in Fig. 7b . Both the traces in Fig. 7b are at the same sweep rate (120 μT s −1 ). By applying a parallel field of 500 mT, we have eliminated the effect of the magnetization dynamics in the ferromagnet. The sharp dips in resistance vanish completely, and only a small positive MR due to weak localization remains. The shift in zero of the H || =500 mT curve is due to the small misalignment of the sample as discussed above. Insulating state I – V characteristics The I – V characteristics of the system were discussed in ref. 8 . The I – V curves in the insulating state were almost linear with no clear evidence of a Coulomb gap, indicating a weak insulating state. However, if dV / dI ( R S ) is plotted as a function of an applied bias current I dc , a peak in dV / dI is observed at low bias. This is shown in Fig. 8 for V g =−30, −45, −60 and −100 V at T =15 mK. For V g =−30 and −45 V, a dip in dV / dI at zero bias signifies the presence of some superconductivity; however, no evidence for that is seen in the temperature dependence of the resistance, as dR / dT <0 at all temperatures in the temperature range of the current experiments. The dip in dV / dI probably arises due to localized superconducting islands weakly phase coupled by the Josephson effect. For V g =−60 and −100 V, the system is in the insulating regime with a peak in dV / dI at zero bias. 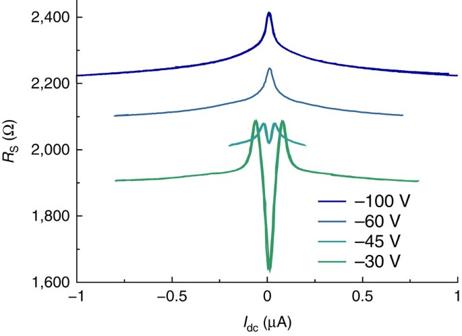Figure 8 Insulating stateI–Vcharacteristics;RSversusIdcfor different gate voltages atT=15 mK. Figure 8 Insulating state I – V characteristics; R S versus I dc for different gate voltages at T =15 mK. Full size image How to cite this article: Mehta, M.M. et al . Evidence for charge–vortex duality at the LaAlO 3 /SrTiO 3 interface. Nat. Commun. 3:955 doi: 10.1038/ncomms1959 (2012).